HACE1-dependent protein degradation provides cardiac protection in response to haemodynamic stress The HECT E3 ubiquitin ligase HACE1 is a tumour suppressor known to regulate Rac1 activity under stress conditions. HACE1 is increased in the serum of patients with heart failure. Here we show that HACE1 protects the heart under pressure stress by controlling protein degradation. Hace1 deficiency in mice results in accelerated heart failure and increased mortality under haemodynamic stress. Hearts from Hace1 −/− mice display abnormal cardiac hypertrophy, left ventricular dysfunction, accumulation of LC3, p62 and ubiquitinated proteins enriched for cytoskeletal species, indicating impaired autophagy. Our data suggest that HACE1 mediates p62-dependent selective autophagic turnover of ubiquitinated proteins by its ankyrin repeat domain through protein–protein interaction, which is independent of its E3 ligase activity. This would classify HACE1 as a dual-function E3 ligase. Our finding that HACE1 has a protective function in the heart in response to haemodynamic stress suggests that HACE1 may be a potential diagnostic and therapeutic target for heart disease. Heart disease is a major cause of death in the developed world, and protection against heart failure is a major challenge [1] . Animal models have shown that inappropriate responses of the heart to sustained haemodynamic stress can lead to heart failure [2] , [3] , [4] . Protein degradation pathways, including the proteasome and autophagy, play a protective role in the response to stress, and their dysregulation appears to underline multiple forms of myocardial disease [5] , [6] , [7] , [8] , [9] , [10] . In post-mitotic cells such as cardiomyocytes, turnover of proteins and organelles is particularly important for cellular protein quality control and maintenance. Two major pathways within the cell that regulate proteolysis are the ubiquitin (Ub)–proteasome system (UPS) and the autophagy lysosomal pathway [6] . Whereas the UPS is mainly involved in the rapid degradation of signalling proteins with short half-lives, autophagy can selectively remove more persistent protein aggregates and damaged organelles [5] . Both proteasome-mediated degradation and selective autophagy require ubiquitination of the cargo, which is then recognized by Ub receptors directing it to either 26S proteasomes or lysosome for degradation [6] . HACE1, as a novel stress inducible Ub E3 protein ligase, has potential roles in both proteolytic systems. We and others previously reported that HACE1 is involved in proteasome-mediated protein degradation [11] , [12] , [13] , [14] , [15] , [16] , [17] . However, HACE1’s involvement in autophagy-mediated protein degradation has never been explored. Increases in autophagic flux have been documented in virtually all forms of human cardiovascular disease, including ventricular hypertrophy and heart failure [18] , [19] . This is indicative of a requirement for autophagy in the maintenance of cellular homoeostasis during ventricular hypertrophic remodelling. Although HACE1 is highly expressed in the heart, nothing is known about its function in the heart. The emerging role of other E3 ligase and Ub-binding proteins in selective autophagy suggests that HACE1 may also participate in this process. Here we demonstrate for the first time that HACE1 is essential for the completion of selective autophagic flux. Hace1 deficiency results in increased accumulation of ubiquitinated protein aggregates in stressed myocardium due to impaired autophagy and thus accelerates cardiac dysfunction. HACE1 is upregulated in human heart failure To clarify the role of HACE1 in the development of heart failure, we performed in silico GEO profiles’ analysis of HACE1 gene expression related to human heart disease. Our search indicated that HACE1 gene expression is upregulated in dilated cardiomyopathy (DCM) compared with non-failing hearts (GEO accession code GDS2206). To confirm this, we examined HACE1 messenger RNA expression in a panel of heart tissue biopsies from heart failure patients as well as non-failing heart controls. Significantly, increased HACE1 gene expression was detected in cardiac tissues of heart failure patients compared with non-failing hearts; there was a 2.5-fold increase in HACE1 gene expression in ischaemic cardiomyopathy and more than a 3-fold increase in DCM ( Fig. 1a ). In addition, markedly elevated Hace1 gene expression was detected in a murine model of heart failure induced by severe transverse aortic constriction (sTAC) compared with a sham-operated control group at 4 days post operation (unpaired two-tailed Student’s t -test, P= 0.0004; Fig. 1b ). The robust induction of HACE1 expression in the heart under pathological stress conditions suggests that HACE1 participates in stress-induced cardiac hypertrophic remodelling. 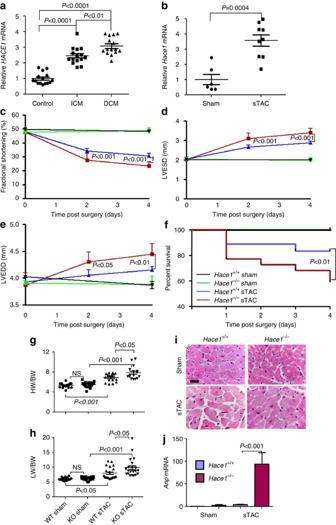Figure 1: Hace1 deficiency accelerates pressure overload-induced heart failure. (a)HACE1mRNA expression is markedly increased in ischaemic and dilated cardiomyopathy (ICM and DCM) heart failure (HF) patient heart tissue compared with non-failing hearts (NF). Expression levels were normalized toHPRTandGAPDHmRNAs.n=15 per group. Control, non-failing heart. (b) ElevatedHace1mRNA expression in sTAC mouse hearts compared with sham controls, expression levels were normalized toHprtandGapdhmRNAs.n=6–9 per group,P=0.004 (unpaired two-tailed Student’st-tests). (c–j)Hace1−/−and WT mice were subjected to sTAC or sham surgery and analysed 4 days after the operation. (c–e) Echocardiographic measurement of (c) LV fractional shortening (FS=(LVEDD−LVESD)/LVEDD × 100%); (d) LV end-diastolic dimension (LVEDD) (mm) and (e) LV end-systolic dimension (LVESD) (mm) are shown.n=6–8 for each group. (f) Mortality rate of WT andHace1−/−mice after sTAC is shown by Kaplan–Meier plots as the survival proportion of each cohort of mice. Survival incidence in mice over the indicated follow-up period is shown as the ratio of the number of mice survived/total mice analysed for each group. This represents 60% (12/20) forHace1−/−sTAC mice, 84% (16/19) forHace1+/+sTAC mice and 100% (12/12) for bothHace1−/−and Hace1+/+sham mice on day 4;Pvalue as indicated (log-rankχ2-test). (g) Heart weight/body weight ratios (HW/BW) and (h) lung weight/body weight ratio (LW/BW) of WT andHace1−/−mice 4 days after sTAC or sham surgery.n=15–21 for each group. (i) Representative haematoxylin and eosin staining transverse heart cross-sections showing myocyte cross-sectional area (scale bars, 20 μm). (j) Real-time RT–PCR analyses reveal a significant increase in the expression of the atrial natriuretic peptide gene (Nppa), a clinical biomarker for heart hypertrophy, inHace1−/−sTAC heart; expression levels were normalized toHprtandGapdhmRNAs.n=6–9 per group. In all panels, error bars represent s.e.m., one-way analysis of variance were used to calculateP-values. Figure 1: Hace1 deficiency accelerates pressure overload-induced heart failure. ( a ) HACE1 mRNA expression is markedly increased in ischaemic and dilated cardiomyopathy (ICM and DCM) heart failure (HF) patient heart tissue compared with non-failing hearts (NF). Expression levels were normalized to HPRT and GAPDH mRNAs. n =15 per group. Control, non-failing heart. ( b ) Elevated Hace1 mRNA expression in sTAC mouse hearts compared with sham controls, expression levels were normalized to Hprt and Gapdh mRNAs. n =6–9 per group, P =0.004 (unpaired two-tailed Student’s t -tests). ( c – j ) Hace1 −/− and WT mice were subjected to sTAC or sham surgery and analysed 4 days after the operation. ( c – e ) Echocardiographic measurement of ( c ) LV fractional shortening (FS=(LVEDD−LVESD)/LVEDD × 100%); ( d ) LV end-diastolic dimension (LVEDD) (mm) and ( e ) LV end-systolic dimension (LVESD) (mm) are shown. n =6–8 for each group. ( f ) Mortality rate of WT and Hace1 −/− mice after sTAC is shown by Kaplan–Meier plots as the survival proportion of each cohort of mice. Survival incidence in mice over the indicated follow-up period is shown as the ratio of the number of mice survived/total mice analysed for each group. This represents 60% (12/20) for Hace1 −/− sTAC mice, 84% (16/19) for Hace1 +/+ sTAC mice and 100% (12/12) for both Hace1 −/− and Hace1 +/+ sham mice on day 4; P value as indicated (log-rank χ 2 -test). ( g ) Heart weight/body weight ratios (HW/BW) and ( h ) lung weight/body weight ratio (LW/BW) of WT and Hace1 −/− mice 4 days after sTAC or sham surgery. n =15–21 for each group. ( i ) Representative haematoxylin and eosin staining transverse heart cross-sections showing myocyte cross-sectional area (scale bars, 20 μm). ( j ) Real-time RT–PCR analyses reveal a significant increase in the expression of the atrial natriuretic peptide gene ( Nppa ), a clinical biomarker for heart hypertrophy, in Hace1 −/− sTAC heart; expression levels were normalized to Hprt and Gapdh mRNAs. n =6–9 per group. In all panels, error bars represent s.e.m., one-way analysis of variance were used to calculate P -values. Full size image Loss of Hace1 accelerates load-induced heart failure in mice Surgical models of cardiac pressure overload in mice have provided a platform for studying load-induced heart failure. To investigate Hace1’s role in the progression of heart failure, we subjected Hace1 −/− and Hace1 +/+ mice to hypertrophic heart failure induced by sTAC [20] . Sham-operated mice were used as controls. Starting from the second day after surgery, noticeable signs of circulatory failure, including lethargy, impaired mobility, diminished appetite and peripheral oedema were observed in mice subjected to sTAC. Echocardiographic measurements revealed no cardiac physiological functional differences between Hace1 −/− , Hace1 +/+ or sham-operated mice at baseline ( Fig. 1c–e ). However, pressure overload induced by sTAC triggers dramatic decreases in left ventricular (LV) function as measured by echocardiography at days 2 and 4 post operation ( Fig. 1c–e ). More importantly, these signs of LV dysfunction were more notable in the Hace1 −/− sTAC-treated mice as shown by a significantly decreased percentage of LV fractional shortening and severely dilated LV, which was indicated by a significant increase in both LV end-diastolic dimension and LV end-systolic dimension compared with wild-type (WT) mice with the same treatment ( Fig. 1c–e ). Moreover, The LV dysfunction resulted in significantly higher mortality rates in Hace1 −/− mice following sTAC; 40% (8/20) of Hace1 −/− mice died between day 1 and day 4 post sTAC, compared with only 16% (3/19) of the Hace1 +/+ mice (log-rank χ 2 -test, P <0.001; Fig. 1f ). This was accompanied by a significant increase in cardiac mass as measured by growing heart weight/body weight ratio in Hace1 −/− sTAC mice compared with Hace1 +/+ sTAC mice ( Fig. 1g ). An increase in myocyte cross-sectional area, as revealed by haematoxylin and eosin staining of left ventricle cross-sections, confirmed that the increase in heart weight/body weight ratio in Hace1 −/− sTAC mice was caused by myocyte enlargement ( Fig. 1i ). Consistent with severe heart failure, Hace1 −/− sTAC mice also had a significantly higher lung weight/body weight ratio, accompanied by pulmonary oedema, compared with Hace1 +/+ sTAC mice ( Fig. 1h ). Expression of atrial natriuretic peptide precursor A, a biomarker of cardiac stress and hypertrophy [21] , [22] , [23] , was also elevated in Hace1 −/− sTAC hearts ( Fig. 1j ). In addition, in our initial pilot studies of HACE1 protein level changes in human clinical plasma samples with heart failure, we also observed some degree of correlation between HACE1 and B-type natriuretic peptide ( Supplementary Fig. 1 ). However, the data only explain 19.5% of the relationship (as per R 2 value), and thus HACE1 and B-type natriuretic peptide do ultimately reflect different biological processes. These findings indicate that, in the absence of Hace1, haemodynamic stress induced by sTAC triggers rapid decompensated cardiac hypertrophic remodelling, progressing to heart failure and increased mortality in these mice. Accumulation of protein aggregates in Hace1 −/− sTAC myocardium To explore Hace1’s role in controlling cardiac remodelling at the cellular level, LV sections of sTAC mice were subjected to transmission electron microscopy (TEM) examination. Ultrastructural analysis of Hace1 −/− sTAC hearts showed a disorganized sarcomere structure and significantly more structures resembling autophagic vacuoles ( Supplementary Fig. 2a ). It is noteworthy that these cellular phenotypes are similar to those previously observed in Atg5-deficient hearts, which are defective in protein/organelle turnover via autophagy [5] . We also observed fewer high-density autolysosome structures in Hace1 −/− sTAC hearts when compared with Hace1 +/+ sTAC hearts ( Supplementary Fig. 2a,b ). In contrast, we observed enlarged autophagosome-like vacuole structures, in some cases containing intact mitochondria, suggesting a disruption in the completion of the autophagy pathway ( Supplementary Fig. 2a ). Ventricular sections from sham-treated Hace1 +/+ and Hace1 −/− mice appeared normal ( Supplementary Fig. 2c,d ). Thus, Hace1 deficiency results in extensive cellular defects in the myocardium during haemodynamic stress. One of the impacts of impaired protein degradation pathways is the accumulation of ubiquitinated proteins [5] , [24] . Immunohistochemical staining of left ventricle cross-sections of sTAC mice revealed a significantly increased accumulation of ubiquitinated proteins in Hace1 −/− myocardium ( Fig. 2a ). This was further confirmed by western blot analysis ( Fig. 2d,e ). The Ub and microtubule-associated protein 1 light chain 3B (LC3II) binding protein p62 (also known as sequestosome 1), which is known to be degraded by autophagy, also accumulates during impairment of autophagy [24] . We observed by immunohistochemical analysis ( Fig. 2b ) and western blot ( Fig. 2d,f ) increased levels of p62 protein in the Hace1 −/− sTAC heart tissue. This suggests that autophagic degradation of p62 was blocked in the absence of Hace1, resulting in the increased cellular accumulation of p62. 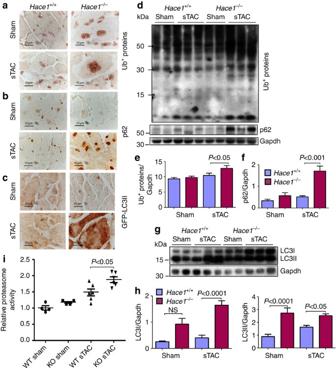Figure 2: Accumulation of p62 LC3 and Ub+protein inHace1−/−sTAC hearts. Representative immunohistochemical staining for (a) ubiquitinated protein (brown); (b) p62 (brown) and (c) GFP-LC3 (brown) in paraffin sections of heart revealing increased accumulation of p62, ubiquitinated protein and LC3 inHace1−/−sTAC hearts. Hearts from three mice in each group were analysed (scale bars, 10 μm). Representative immunoblot and quantification for (d,e) Ub-conjugated proteins, (d,f) p62 and (g,h) LC3 in heart extracts (n=3 per group), Gapdh were used as a loading control. (i) Increased Ub proteasome activity inHace1−/−sTAC hearts as measured by 20S proteasome activity assay (n=4–6 per group). In all panels, error bars represent s.e.m.,Pvalue between KO and WT sTAC as indicated (one-way analysis of variance). Figure 2: Accumulation of p62 LC3 and Ub + protein in Hace1 −/− sTAC hearts. Representative immunohistochemical staining for ( a ) ubiquitinated protein (brown); ( b ) p62 (brown) and ( c ) GFP-LC3 (brown) in paraffin sections of heart revealing increased accumulation of p62, ubiquitinated protein and LC3 in Hace1 −/− sTAC hearts. Hearts from three mice in each group were analysed (scale bars, 10 μm). Representative immunoblot and quantification for ( d , e ) Ub-conjugated proteins, ( d , f ) p62 and ( g , h ) LC3 in heart extracts ( n =3 per group), Gapdh were used as a loading control. ( i ) Increased Ub proteasome activity in Hace1 −/− sTAC hearts as measured by 20S proteasome activity assay ( n =4–6 per group). In all panels, error bars represent s.e.m., P value between KO and WT sTAC as indicated (one-way analysis of variance). Full size image Next, we assessed autophagy by examining microtubule-associated protein LC3, an autophagy protein that is present in the cytosol (LC3-I form) until it becomes targeted to nascent autophagosomes via conjugation to phosphatidylethanoloamine (LC3-II form) [25] . Levels of LC3 were first examined by western blot ( Fig. 2c,g ). In Hace1 −/− sTAC hearts, we observed a significant increase in total LC3 protein levels. Both LC3-I and the LC3-II forms of the protein accumulated to a significantly higher level in Hace1 −/− sTAC hearts when compared with Hace1 +/+ controls. Enhanced LC3 accumulation was also observed in Hace1 −/− / LC3 Tg sTAC myocardium, which stably expresses green fluorescence protein (GFP)-LC3 under the β-actin (CAG) promoter [26] ( Fig. 2h ). Moreover, no significant increase in p62 or Lc3b gene expression was detected in Hace1 −/− sTAC heart ( Supplementary Fig. 3 ), suggesting that the increased p62 and LC3 accumulation were due to impaired degradation by autophagy at the post-transcriptional level. It is possible that defects in proteasomal activity were responsible for the ubiquitinated protein accumulation in sTAC Hace1 −/− myocardium. However, heart lysates from sTAC-treated Hace1 −/− mice displayed elevated 20S proteasome levels compared with Hace1 +/+ hearts ( Fig. 2i ). This may reflect a compensating mechanism to overcome the impairment of autophagy. Indeed, elevated cardiac proteasomal activity accompanies autophagy deficiency on deletion of Atg5 (ref. 5 ). Thus, Hace1 deficiency impaired the clearance of ubiquitinated proteins in the myocardium and is associated with the acceleration of heart failure. In addition to its role in protein degradation by the proteasome [11] , [12] , [13] , [14] , [15] , our data indicate that HACE1 is also required for efficient functioning of the autophagy pathway in the heart during haemodynamic stress. HACE1 controls autophagic clearance of protein aggregates To better understand HACE1’s function in the clearance of ubiquitinated proteins under stress conditions, we examined its role in protein aggregate clearance in both primary neonatal cardiomyocytes (NCMs) and embryonic fibroblasts (MEFs) derived from Hace1 −/− and Hace1 +/+ control mice. Ubiquitinated protein aggregate formation was induced by treatment with puromycin, an inhibitor of protein translation that induces premature polypeptide chain termination and the subsequent accumulation of misfolded proteins, which can be detected with a monoclonal antibody specific to ubiquitinated proteins [27] . Immunofluorescence staining shows HACE1 localized to ubiquitinated protein aggregates in puromycin-treated MEF ( Fig. 3a ). This suggests that HACE1 may act locally at the aggregates to promote protein turnover. To test this hypothesis, we subjected WT and Hace1 −/− primary NCMs to an aggregate clearance assay [27] , [28] , where cells were pulsed with puromycin for 4 h to induce protein aggregate formation. The treatment was then removed by extensive washing, followed by an 8-h chase to allow for aggregate clearance. The majority of WT NCM was able to clear aggregates by 8 h after puromycin removal ( Fig. 3b ). In contrast, aggregate clearance was almost completely blocked in Hace1 −/− NCM. 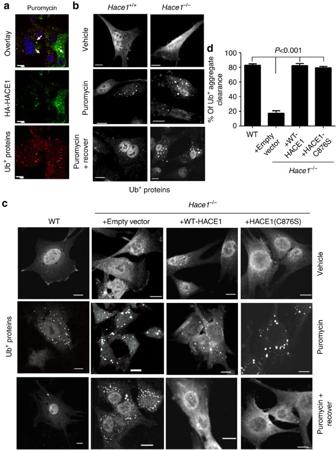Figure 3: HACE1 is required for autophagic clearance of Ub+protein aggregates independent of its E3 ligase activity. (a) Representative confocal microscopy images showing HACE1 (green) localizing to the Ub+protein aggregates (red) induced by puromycin treatment in HA-HACE1 MEF. Arrows indicate co-localized puncta. Scale bar, 10 μm. (b) Representative confocal micrographs of Hace1−/−and Hace1+/+NCM treated with puromycin for 4 h (puromycin), puromycin followed by 8 h recover (puromycin+recover). Vehicle (PBS)-treated cells were used as control. Hace1 deficiency in cardiomyocytes (Hace1−/−NCM) blocks ubiquitinated protein aggregate degradation. Scale bars, 10 μm. (c,d) WT and Hace1−/−MEF as well as Hace1−/−MEF stably transfected with WT HACE1 and C876S-mutant HACE1were subjected to protein aggregates clearance assay by pulsing with puromycin for 4 h to induce protein aggregate formation followed by an 8-h chase to monitor for aggregate clearance. Cells were fixed and stained for ubiquitinated proteins to visualize aggregates. Vehicle (PBS)-treated MEFs were used as control. (c) Representative confocal micrographs of images used for quantification of the efficiency of aggregates clearance ind(percentage of cells that cleared all aggregates by 8 h after puromycin removal). At least 10 images from each group were used for the calculation, error bars represent s.e.m.,P<0.001 (one-way analysis of variance). Scale bars, 10 μm. Figure 3: HACE1 is required for autophagic clearance of Ub + protein aggregates independent of its E3 ligase activity. ( a ) Representative confocal microscopy images showing HACE1 (green) localizing to the Ub + protein aggregates (red) induced by puromycin treatment in HA-HACE1 MEF. Arrows indicate co-localized puncta. Scale bar, 10 μm. ( b ) Representative confocal micrographs of Hace1 −/− and Hace1 +/+ NCM treated with puromycin for 4 h (puromycin), puromycin followed by 8 h recover (puromycin+recover). Vehicle (PBS)-treated cells were used as control. Hace1 deficiency in cardiomyocytes (Hace1 −/− NCM) blocks ubiquitinated protein aggregate degradation. Scale bars, 10 μm. ( c , d ) WT and Hace1 −/− MEF as well as Hace1 −/− MEF stably transfected with WT HACE1 and C876S-mutant HACE1were subjected to protein aggregates clearance assay by pulsing with puromycin for 4 h to induce protein aggregate formation followed by an 8-h chase to monitor for aggregate clearance. Cells were fixed and stained for ubiquitinated proteins to visualize aggregates. Vehicle (PBS)-treated MEFs were used as control. ( c ) Representative confocal micrographs of images used for quantification of the efficiency of aggregates clearance in d (percentage of cells that cleared all aggregates by 8 h after puromycin removal). At least 10 images from each group were used for the calculation, error bars represent s.e.m., P <0.001 (one-way analysis of variance). Scale bars, 10 μm. Full size image To evaluate whether HACE1’s E3 ligase activity is required for the clearance of protein aggregates, we next compared the effects of WT and mutant HACE1 expression on rescue of aggregate clearance. Hace1 −/− MEF stably transfected with either WT HACE1 complementary DNA ( WT-HACE1 ) or a C876S point mutated form of HACE1 (C876S) were used for the rescue studies. The point mutation of amino acid 876 from cysteine to serine is known to abolish E3 ligase activity of HACE1 (refs 11 , 12 , 13 , 14 , 15 ). As expected, the defects in aggregate clearance in Hace1 −/− MEF were rescued by WT HACE1. Surprisingly, HACE1 (C876S) rescued the protein aggregate clearance defect as efficiently as WT HACE1 ( Fig. 3c,d ). ANK domain in HACE1 is required for removal of protein aggregates To date, the only known HACE1 E3 ligase substrate is Rac1. It has been shown that HACE1 controls Rac1 activity through binding and ubiquitinating the GTP-bound form of Rac1, leading to its proteasomal degradation [13] , [14] , [15] . Transgenic mice overexpressing Rac1 exhibit the phenotype of cardiac hypertrophy and DCM [29] . To test the possibility that upregulated Rac1 may contribute to the heart failure phenotype in Hace1 −/− sTAC mice, we subjected sTAC hearts to Rac1 immunoblotting. 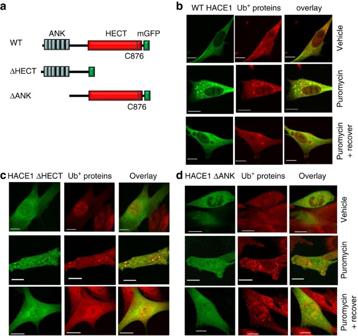Figure 4: ANK domain in HACE1 is necessary for autophagic removal of Ub+protein aggregates. (a) Diagrams representing GFP-tagged WT HACE1 and mutant HACE1 (HACE1Δ HECT and HACE1Δ ANK) constructs transiently transfected intoHace1−/−MEF for protein aggregate clearance assay. (b–d) Representative confocal micrographs of (b) WT, (c) ΔHECT and (d) ΔANK MEF subjected to protein aggregate clearance assay by pulsing with puromycin for 4 h to induce protein aggregate formation followed by an 8-h chase to monitor for aggregate clearance. Vehicle-treated MEFs were used as control. Scale bars, 10 μm. No significant changes in Rac1 protein levels were detected between Hace1 −/− and WT groups ( Supplementary Fig 4a ). Although we cannot exclude the possibility that Rac1 may participate in the cardiac remodelling process under stress, at least in the particular experimental settings that we have tested, Rac1 does not appear to be regulated by Hace1. A report by Zhao et al. [17] indicated that HACE1 is a novel repressor of retinoic acid receptor (RAR) transcription, a role that is independent from its E3 Ub ligase activity. This suggests that HACE1 has additional function(s) beyond its role as an E3 Ub ligase. To explore this further, we subjected sTAC hearts to RAR-β immunoblotting. We detected no significant changes in RAR-β protein levels between Hace1 −/− and WT groups ( Supplementary Fig 4b ). This suggests that RAR-β did not significantly contribute to the heart failure phenotype in the Hace1 −/− sTAC mice. Besides the HECT domain, the other known domain of HACE1 is the six ankyrin repeats (ANK) at its amino terminal. However, the function of the ANK domain in HACE1 is entirely unknown. On the basis of our finding that HACE1 promotes ubiquitinated protein aggregate clearance independently of its E3 ligase activity, we hypothesize that HACE1 functions as an adaptor protein, binding to ubiquitinated proteins and delivering them for autophagic degradation via HACE1’s ANK domain. To test this hypothesis, three GFP-tagged HACE1 plasmids, WT HACE1-GFP, HACE1ΔHECT-mGFP and HACE1ΔANK-mGFP , were generated. The two mutant HACE1 constructs were generated by DNA synthesis with deletion of either the carboxy-terminal HECT domain (ΔHECT) or the N-terminal ANK repeat (ΔANK; Fig. 4a ). After transient transfection of the plasmid into Hace1 −/− MEF, MEF were subjected to a protein aggregate clearance assay. Similar to WT HACE1 ( Fig. 4b ), HACE1Δ HECT localized to ubiquitinated protein aggregates in puromycin-treated MEF. Moreover, similar to WT HACE1, the majority of HACE1Δ HECT cells were able to clear aggregates by 8 h after puromycin removal ( Fig. 4c ). In contrast, HACE1ΔANK did not localize with ubiquitinated protein aggregates and lost the ability to clear aggregates after puromycin removal ( Fig. 4d ). Therefore, HACE1 is required for efficient clearance of protein aggregates and this is independent of its E3 ligase activity. Instead, HACE1 may participate in the delivery of ubiquitinated protein aggregates to the autophagic lysosomal pathway for degradation via protein–protein interactions mediated by its ANK domain. Figure 4: ANK domain in HACE1 is necessary for autophagic removal of Ub + protein aggregates. ( a ) Diagrams representing GFP-tagged WT HACE1 and mutant HACE1 (HACE1Δ HECT and HACE1Δ ANK) constructs transiently transfected into Hace1 −/− MEF for protein aggregate clearance assay. ( b – d ) Representative confocal micrographs of ( b ) WT, ( c ) ΔHECT and ( d ) ΔANK MEF subjected to protein aggregate clearance assay by pulsing with puromycin for 4 h to induce protein aggregate formation followed by an 8-h chase to monitor for aggregate clearance. Vehicle-treated MEFs were used as control. Scale bars, 10 μm. Full size image HACE1 partners with p62 in protein aggregate clearance The adaptor protein p62 has the ability to bind to both ubiquitinated proteins and LC3II (ref. 30 ). In the Hace1 −/− sTAC heart, we observed a significant increase in p62-positive puncta ( Fig. 2d ). To determine whether HACE1 co-localized with p62, Hace1 −/− NCM transiently expressing HACE1-GFP were subjected to p62 immunofluorescent staining. Under control conditions, HACE1 expressed uniformly across the cytoplasm, mostly not localizing with p62. However, on puromycin treatment, both HACE1 and p62 relocated to the perinuclear region and, more importantly, co-localized ( Fig. 5a ). This indicates that HACE1 may control protein aggregate degradation via regulation of p62. To further address whether HACE1 partners with p62 in protein aggregate clearance, we depleted p62 by short interfering RNA (siRNA) in Hace1 +/+ and Hace1 −/− MEFs ( Supplementary Fig. 5a ) and subjected cells to a protein aggregate clearance assay. Knockdown of p62 partially restored ubiquitinated protein aggregate degradation in Hace1 −/− MEF ( Supplementary Fig. 5b ), suggesting p62 could be a downstream target of HACE1. It has been reported that p62 promotes the formation of polyubiquitinated protein aggregates to allow clearance via autophagy [24] , [30] , [31] . Therefore, in HACE1 knock-out cells, where autophagy is impaired, p62 knockdown would inhibit aggregate formation but presumably not total cellular ubiquitination and toxicity. To test whether E3 Ub ligase activity is involved in HACE1’s interaction with p62, WT, Hace1 −/− MEFs and Hace1 −/− MEF stably transfected with either WT HACE1 ( WT-HACE1 ) or a C876S-mutant form HACE1(C876S) were treated with MG132, a specific, potent and cell permeable proteasome inhibitor that reduces the degradation of Ub-conjugated proteins in mammalian cells [32] , [33] , [34] , [35] , for 4 h to induce ubiquitinated protein aggregates formation. When p62-immunoprecipitated samples were subjected to immunobloting with FK2 (Ub-conjugated proteins) antibody, we observed increased Ub-conjugated proteins in Hace1 −/− MEF. 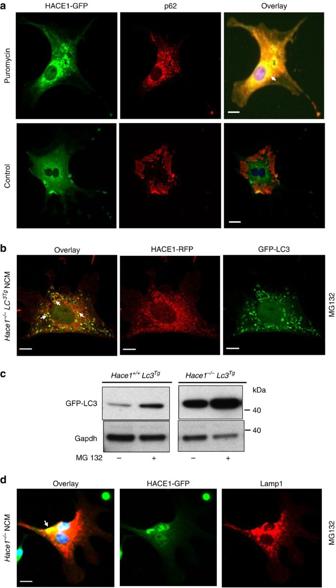Figure 5: HACE1 contributes to autophagic clearance of protein aggregates in a p62-dependent manner. (a) Fluorescence microscopy images showing HACE1 (green) co-aggregating with p62 (red) in the perinuclear space on puromycin treatment (8 h) inHace1−/−NCM transiently expressing HACE1-GFP. p62 was visualized by immunofluorescent staining. Arrows indicate co-localized puncta. (b) Representative confocal images showing HACE1 (red) localizes to LC3+puncta (green) induced by MG132 treatment (8 h) inHace1−/−GFP-Lc3TgNCM cells transiently expressing HACE1-RFP. Arrows indicate co-localized puncta. (c) Primary NCMs fromHace1+/+Lc3TgandHace1−/−Lc3Tgnewborn pups were treated with or without MG132 for 8 h and the cell lysates were subjected to western blot with anti-GFP antibodies. Gapdh was used as a loading control. (d) Fluorescence microscopy images showing co-localization of HACE1 (green) with Lamp1 (red) on MG132 treatment (8 h) inHace1−/−NCM cells transiently expressing HACE1-GFP. Lamp1 was visualized by immunofluorescent staining. Scale bar, 10 μm in all images. Adding either WT or C876S mutant back to Hace1 −/− MEF decreased the pull-down of UB-conjugated proteins to a similar level as WT ( Supplementary Fig 5c ). Our data indicate that HACE1 expression can affect p62 levels independently of its E3 Ub ligase activity. Therefore, HACE1 may serve as an adaptor for autophagy in addition to its role in protein degradation via the Ub–proteasome pathway. Figure 5: HACE1 contributes to autophagic clearance of protein aggregates in a p62-dependent manner. ( a ) Fluorescence microscopy images showing HACE1 (green) co-aggregating with p62 (red) in the perinuclear space on puromycin treatment (8 h) in Hace1 −/− NCM transiently expressing HACE1-GFP. p62 was visualized by immunofluorescent staining. Arrows indicate co-localized puncta. ( b ) Representative confocal images showing HACE1 (red) localizes to LC3 + puncta (green) induced by MG132 treatment (8 h) in Hace1 −/− GFP-Lc3 Tg NCM cells transiently expressing HACE1-RFP. Arrows indicate co-localized puncta. ( c ) Primary NCMs from Hace1 +/+ Lc3 Tg and Hace1 −/− Lc3 Tg newborn pups were treated with or without MG132 for 8 h and the cell lysates were subjected to western blot with anti-GFP antibodies. Gapdh was used as a loading control. ( d ) Fluorescence microscopy images showing co-localization of HACE1 (green) with Lamp1 (red) on MG132 treatment (8 h) in Hace1 −/− NCM cells transiently expressing HACE1-GFP. Lamp1 was visualized by immunofluorescent staining. Scale bar, 10 μm in all images. Full size image HACE1 is required for the completion of autophagic flux The above findings are consistent with the notion that HACE1 is a novel potential regulator of the selective autophagy pathway. Next, we tried to determine in which step of autophagy HACE1 participates. Changes in gene expression from a panel of autophagy-related genes were analysed by quantitative PCR in sTAC and sham hearts. We found no significant differences in expression between WT and Hace1 −/− sTAC hearts in genes related to autophagy initiation such as Atg5, Atg7 and Beclin1 ( Supplementary Fig. 6 ). This indicates that the induction phase of autophagy is not affected by Hace1 deficiency. Autophagy is a dynamic process with autophagosome formation being balanced by turnover on delivery to lysosomes. Inhibition of lysosome-mediated degradation will block LC3 degradation and hence increase LC3 accumulation [20] . Enhanced LC3 accumulation in Hace1 −/− sTAC heart ( Fig. 2h ) suggests that HACE1 deficiency could block autophagic flux. To verify this, HACE1’s interaction with LC3 was examined in Hace1 −/− /GFP- LC3 Tg NCM transiently expressing HACE1-RFP. Blockade of UPS by proteasome inhibition has been shown to activate autophagy [32] , [33] , [34] , [35] . Exposure of the NCM to MG132 led to the co-localization of HACE1 with LC3 puncta ( Fig. 5b ). In addition, when we subjected MG132-treated Hace1 −/− /GFP- LC3 Tg NCM and control Hace1 +/+ /GFP- LC3 Tg NCM cells to LC3 immunoblot analysis, HACE1 deficiency clearly led to increased GFP-LC3 accumulation in Hace1 −/− /GFP- LC3 Tg NCM compared with WT control ( Fig. 5c ). This suggests that lysosome-mediated degradation is impaired in the absence of HACE1. Indeed, HACE1-GFP-labelled structures also co-localized with the lysosomal marker, Lamp1 ( Fig. 5d ), suggesting that HACE1 may be required for autolysosome formation. To determine whether HACE1 is required for the fusion of autophagosomes with lysosomes, we used a tandem tagged mRFP-GFP-LC3 (tfLC3) probe. This probe can be used to detect whether an autophagosome has fused with a lysosome, based on the distinct chemical properties of GFP and mRFP fluorophores. Under neutral pH conditions in the cytosol, both GFP and mRFP moieties of the probe fluoresce. However, under low pH conditions in the lumen of the lysosome, the GFP signal is quenched, but not the mRFP. By exploiting the difference in the nature of these two fluorescent proteins, autophagic flux can be measured with this mRFP-GFP-LC3 tandem probe [36] . First, we tested the tfLC3 reporter in WT and Hace1 −/− primary NCMs 48 h after transient transfection with tfLC3 plasmid. NCM were treated with MG132 for 8 h to induce autophagy, as previously described [34] . In addition, bafilomycin A1 (Baf), an inhibitor of lysosomal acidification, was added to one of the MG132-treated groups in the last 4 h to inhibit autolysosome formation. MG132 is capable of inducing autophagy in WT and Hace1 −/− NCM, as measured by increased GFP-LC3-positive puncta compared with the untreated group ( Fig. 6a ). However, fewer green/red autophagosomes and more red-only autolysosomes were detected in MG132-treated Hace1 WT NCM, and treatment with Baf reversed this pattern. In contrast, loss of Hace1 resulted in a significant increase in green/red-positive autophagosome structures with a reduction in red-only autolysosome structures in the absence of Baf as shown in Hace1 −/− NCM. In addition, no significant changes were observed in Hace1 −/− NCM co-treated with Baf ( Fig. 6a,b ). This indicates that there is a defect in autophagosome–lysosome fusion in Hace1-deficient cardiomyocytes. To test whether the E3 ligase activity of Hace1, if required for this process, we next tested the tfLC3 reporter in Hace1 −/− MEF stably transfected with empty vector ( MSCV ), WT HACE1 ( HA-HACE1 ) and E3 ligase dead HACE1 ( C876S-HACE1 ). WT MEF was used as a control. After 4 h incubation with MG132, WT MEF had fewer green/red autophagosomes and more red autolysosomes; in contrast, significantly increased green/red-positive autophagosome structures and reduced red-positive-only autolysosome structures were observed in Hace1 −/− ( MSCV ) MEF. As expected, the defects in autophagosome–lysosome fusion in Hace1 −/− MEF were rescued by WT HACE1. Moreover, E3 ligase mutation in HACE1 (C876S MEF cells) results in similar mRFP-GFP-LC3 expression patterns as WT ( Fig. 6c,d ). This suggests that HACE1 is required for the fusion of autophagosomes with lysosomes independent of its E3 ligase activity. 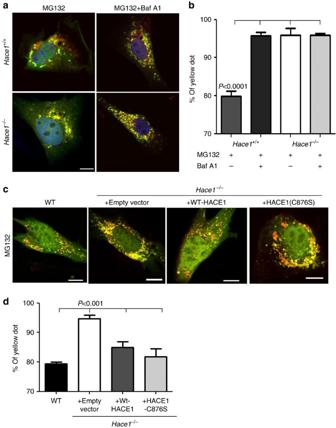Figure 6: Hace1 is essential for the completion of autophagic flux. (a,b) Primary NCMs from WT andHace1−/−newborn pups and (c,d) WT andHace1−/−MEF, as well asHace1−/−MEF stably transfected with WT HACE1 and C876S-mutant HACE1, were transiently transfected with a tandem tagged mRFP-GFP-LC3 reporter (tfLC3) plasmid, followed by 8 h treatment with MG132 or MG132 plus Baf in the last 4 h, and were subjected to confocal microscopy. DMSO treatment only was used in the control group. (a,c) Representative confocal micrographs of images used for quantification of the percentage of yellow dots inbandd. At least 10 images from each group were used for the calculation; error bars represent s.e.m.,P-value as indicated (one-way ANAVO). Scale bars, 10 μm. Autophagosomes show both GFP and mRFP-LC3 signals (yellow) while autolysosomes exhibit mRFP-L3 signals only (red). Figure 6: Hace1 is essential for the completion of autophagic flux. ( a , b ) Primary NCMs from WT and Hace1 −/− newborn pups and ( c , d ) WT and Hace1 −/− MEF, as well as Hace1 −/− MEF stably transfected with WT HACE1 and C876S-mutant HACE1, were transiently transfected with a tandem tagged mRFP-GFP-LC3 reporter ( tfLC3 ) plasmid, followed by 8 h treatment with MG132 or MG132 plus Baf in the last 4 h, and were subjected to confocal microscopy. DMSO treatment only was used in the control group. ( a , c ) Representative confocal micrographs of images used for quantification of the percentage of yellow dots in b and d . At least 10 images from each group were used for the calculation; error bars represent s.e.m., P -value as indicated (one-way ANAVO). Scale bars, 10 μm. Autophagosomes show both GFP and mRFP-LC3 signals (yellow) while autolysosomes exhibit mRFP-L3 signals only (red). Full size image HACE1 is required for maintaining protein homoeostasis To identify HACE1-interacting proteins, a combination of co-immunoprecipitation assay (Co-IP) with mass spectrometry (MS) analysis was conducted in Hace1 −/− MEF stably expressing an N-terminal haemagglutinin (HA)-tagged full-length HACE1 protein (HA-HACE1) [12] . Empty vector ( MSCV )-transfected Hace1 −/− MEFs were used as controls. HA-tagged HACE1 protein expression was readily detectable in HA-HACE1 -transfected MEF but not in the empty vector ( MSCV )-transfected MEF ( Fig. 7a ). After resolved by SDS–polyacrylamide gel electrophoresis (PAGE), coomassie blue staining detected several distinct bands in the anti-HA Co-IP pull-down products from HA-HACE1 MEF lysates but not in the control Hace1 −/− MSCV MEF ( Fig. 7b ). The anti-HA Co-IP pull-down products were further subjected to MS analysis. We performed a total of five experimental replicates for HA-HACE1-expressing MEF and four experimental replicates for control Hace1 −/− MSCV-MEF. A total of 173 different proteins were identified from all nine purifications with 158 identified in any of the five HA-HACE1 purifications. To identify potential HACE1 interactors of high confidence, the proteins were filtered by selecting proteins that were found in more than or equal to two HA-HACE1 purifications, and then were found to be at least twofold enriched, by spectral counts, in the HA-HACE1 purification when compared with the control sample. This data reduction yielded 73 potential binding partners ( Fig. 7c and Supplementary Table 1 ). 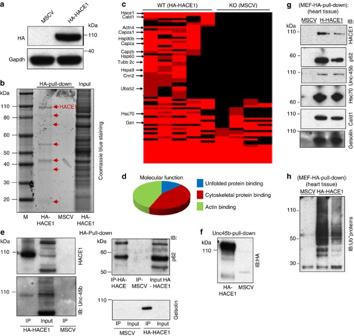Figure 7: Identification of HACE1 interacting proteins by MS analysis of HA Co-IP. (a,b)Hace1−/−MEF cells were stably transfected with HA-tagged WT HACE1 (HA-HACE1) and empty vector MSCV. (a) Immunoblot for HA shows stable expression of HA-tagged HACE1 in HA-HACE1 MEF cell lysate. (b) HA-HACE1 MEF and control MSCV MEF cell lysates were subjected to Co-IP with anti-HA antibody and coomassie blue staining shows a couple of distinct bands only detected in HA-HACE1 MEF IP pull-down as indicated by red arrows. (c–f) Identification of HACE1 interacting proteins by MS analysis of Co-IP products. (c) Hierarchical clustering (heat) map demonstrating the clustering of proteins based on their expression intensities in HA-HACE1 MEF and control MSCV MEF HA-IP pull-down products. To the left of the heat map, selected annotations found to be enriched in the protein clusters are shown.n=5 for HA-HACE1 group andn=4 for control MSCV group. (d) Pie chart shows enriched representative HACE1-interacting proteins according to molecular function by GO term. (e) Selected HACE1-interacting proteins identified by HA-IP MS were evaluated by western blot with the indicated antibodies (IB). HA-HACE1 denotes HA-IP pull-down from HA-HACE1 MEF; MSCV denotes HA-IP pull-down from control MSCV MEF; and input indicates HA-HACE1 MEF lysate before IP. (f) HA-HACE1 MEF and control MSCV MEF lysates were subjected to co-IP with an anti-Unc-45b antibody and the pull-down were analysed by western blot with an anti-HA antibody. (g,h) HA-IP pull-down products from HA-HACE1 MEF (HA-HACE1) andHace1KO MSCV MEF (MSCV) immortalized in HA beads were further subjected to Co-Co-IP with WT mouse heart lysates, and the pull-down products were analysed by western blot using the indicated antibodies. HACE1 and those proteins with which it interacts were still detectable (g). There were also increased ubiquitinated proteins in the Co-Co-IP heart tissues (h). Figure 7: Identification of HACE1 interacting proteins by MS analysis of HA Co-IP. ( a , b ) Hace1 −/− MEF cells were stably transfected with HA-tagged WT HACE1 (HA-HACE1) and empty vector MSCV. ( a ) Immunoblot for HA shows stable expression of HA-tagged HACE1 in HA-HACE1 MEF cell lysate. ( b ) HA-HACE1 MEF and control MSCV MEF cell lysates were subjected to Co-IP with anti-HA antibody and coomassie blue staining shows a couple of distinct bands only detected in HA-HACE1 MEF IP pull-down as indicated by red arrows. ( c – f ) Identification of HACE1 interacting proteins by MS analysis of Co-IP products. ( c ) Hierarchical clustering (heat) map demonstrating the clustering of proteins based on their expression intensities in HA-HACE1 MEF and control MSCV MEF HA-IP pull-down products. To the left of the heat map, selected annotations found to be enriched in the protein clusters are shown. n =5 for HA-HACE1 group and n =4 for control MSCV group. ( d ) Pie chart shows enriched representative HACE1-interacting proteins according to molecular function by GO term. ( e ) Selected HACE1-interacting proteins identified by HA-IP MS were evaluated by western blot with the indicated antibodies (IB). HA-HACE1 denotes HA-IP pull-down from HA-HACE1 MEF; MSCV denotes HA-IP pull-down from control MSCV MEF; and input indicates HA-HACE1 MEF lysate before IP. ( f ) HA-HACE1 MEF and control MSCV MEF lysates were subjected to co-IP with an anti-Unc-45b antibody and the pull-down were analysed by western blot with an anti-HA antibody. ( g , h ) HA-IP pull-down products from HA-HACE1 MEF (HA-HACE1) and Hace1 KO MSCV MEF (MSCV) immortalized in HA beads were further subjected to Co-Co-IP with WT mouse heart lysates, and the pull-down products were analysed by western blot using the indicated antibodies. HACE1 and those proteins with which it interacts were still detectable ( g ). There were also increased ubiquitinated proteins in the Co-Co-IP heart tissues ( h ). Full size image A gene ontology term enrichment analysis was performed to determine which molecular functions and biological processes were over-represented. Gene names corresponding to the 73 proteins found in multiple HA-HACE1 purifications were submitted for statistical enrichment of gene ontology pathway analysis using the Gene Ontology For Functional Analysis software tools in ArrayTrack (ArrayTrack http://www.fda.gov/ScienceResearch/BioinformaticsTools/Arraytrack ) [37] . Terms associated with ‘cytoskeletal binding and organization’, ‘the unfolded protein response’ and ‘protein complex disassembly’ were found to be statistically enriched ( P ≤0.05, n ≥5, E >2, Fisher’s exact test; Fig. 7d ). Among them, several cytoskeletal proteins like gelsolin [38] , Fhl1 (refs 39 , 40 , 41 ) and vinculin [42] , [43] were found to be the important mediators of cardiomyopathy. Western blot analysis confirmed that p62, gelsolin and Unc-45b are among these binding partners of HACE1 ( Fig. 7e ). Moreover, when Co-IP was performed of the same MEF lysate with anti Unc-45b antibody, HA-HACE1 was readily detectable ( Fig. 7f ). In addition, when the HA-HACE1 MEF Co-IP pull-down complex were further bound with whole-heart lysate (Co-Co-IP) from HACE1 WT mice, HACE1 and its interaction proteins p62, Unc-45b, Hsc70, gelsolin and caldesmon 1 were still detectable ( Fig. 7g ). Furthermore, there were also increased ubiquitinated proteins in the Co-Co-IPs from heart tissues ( Fig. 7h ). This indicates that HACE1 is binding to these proteins in the heart in addition to MEF. Accumulation of Hace1 binding partners in Hace1 −/− sTAC heart On the basis of above observations, we predicted that proteins interacting with HACE1 would accumulate in the hearts of sTAC-treated Hace1 −/− mice. We tested whether HACE1 deficiency results in accumulation of those proteins in the stressed myocardium in vivo under haemodynamic stress. We observed significantly increased accumulation of many HACE1-interacting proteins, such as Fhl1, vimentin, Unc-45b, galdesmon 1, β-tubulin ( Fig. 8a,d ), gelsolin and vinculin ( Fig. 8b,d ) in the Hace1 −/− sTAC heart compared with Hace1 +/+ controls. Molecular chaperones Hsp70, Hsc70 and Hsp25 were also significantly accumulated in the Hace1 −/− sTAC heart ( Fig. 8c,d ). In addition, expression levels of control proteins that were not identified in our HACE1 Co-IP assay, like connexin 40 and connexin 43, were not affected by Hace1 deficiency ( Supplementary Fig. 7 ). Thus, HACE1 deficiency leads to the accumulation of its binding partners under haemodynamic stress in the heart. 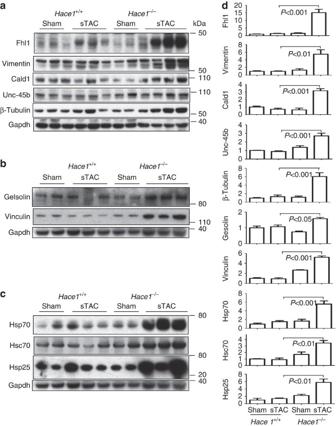Figure 8: Proteins interacting with HACE1 accumulate inHace1−/−sTAC heart. (a–c) Representative western blots and (d) quantification show increased accumulation of some of the HACE1-interacting proteins in theHace1−/−sTAC myocardium.n=3 mice per group, error bars represent s.e.m.,P-value between KO and WT sTAC as indicated (one-way analysis of variance). Gapdh was used as a loading control. Figure 8: Proteins interacting with HACE1 accumulate in Hace1 −/− sTAC heart. ( a – c ) Representative western blots and ( d ) quantification show increased accumulation of some of the HACE1-interacting proteins in the Hace1 −/− sTAC myocardium. n =3 mice per group, error bars represent s.e.m., P -value between KO and WT sTAC as indicated (one-way analysis of variance). Gapdh was used as a loading control. Full size image Levine and colleagues recently demonstrated that the HECT domain E3 ligase SMURF1 promotes degradation of viral capsid proteins independently of its E3 ligase activity but requiring its membrane-binding C2 domain [44] . These authors proposed that the C2 domain of SMURF1 may participate in the delivery of selective autophagic substrates to the nascent autophagosome. In this manner, SMURF1 may participate in both proteasomal degradation (via its E3 ligase activity) and autophagy (via its C2 domain). Both HACE1 and SMURF1 belong to the HECT domain E3 ligase family. The difference is instead of the C2 domain, HACE1 has an ANK repeat domain at its N terminal and the function of this domain in HACE1 has not been explored. We demonstrated here that HACE1, similar to SMURF1, is a dual function E3 ligase that can promote degradation of selective cargo by at least two independent mechanisms that differ in their requirement for E3 ligase activity. HACE1 participates in proteasomal degradation via its HECT domain E3 ligase activity and contributes to autophagic degradation via its ANK domain-mediated protein–protein interactions. Remarkably, the role of HACE1 in cellular proteostasis only becomes apparent under stress. This may indicate that redundant pathways of protein degradation can complement for HACE1 deficiency in the basal state, and that these pathways are impaired or inadequate during cellular stress. Our data indicate that HACE1 deficiency impairs autophagy in the heart during haemodynamic stress. Besides catalysing the ubiquitination of active Rac1 (refs 13 , 14 , 15 ), the roles of HACE1 in mediating Golgi traffic [16] , suppression of RAR signalling [17] and the degradation of specific proteins may underlie this autophagy defect. Many HACE1-interacting proteins are associated with cytoskeletal function. A properly balanced cytoskeletal quality control is essential for cellular and organismal structure and function [45] , [46] , [47] . The maintenance of cardiac cytoskeletal homoeostasis becomes even more essential in the context of disease, where appropriate remodelling is necessary for survival. Cytoskeleton-specific chaperones and Ub ligases are necessary for the assembly and degradation of cytoskeletal proteins and constitute the protein quality control system in the heart [45] . However, very little is known about the actual mechanisms responsible for regulating the turnover of the cardiac cytoskeleton [46] . A recent study suggested that specific Ub E3 protein ligases regulate degradation pathways for actin (via TRIM32) [46] and tubulin (via Parkin) [47] . There is also evidence that the co-chaperones Unc-45 and Hsp90 are required for myosin quality control [4] . In the present study, we found HACE1 physically binding with Unc-45B both by IP and reverse IP ( Fig. 7e–f ). When we subjected the Co-IP products to MS analysis; indeed, proteins associated with cytoskeleton binding and organization and the unfolded protein response and protein complex disassembly were enriched ( Fig. 7c,d ). This suggests that HACE1 may form a complex with Unc-45b, Hsc70, Hsp90 as well as other chaperons and cytoskeletal binding and organization proteins to facilitate the proper organization and turnover of cytoskeletal proteins. Thus, our data suggest that HACE1 is a stress inducible, selective safeguard for cytoskeleton homoeostasis that is required for normal cardiac responses to haemodynamic stress. In conclusion, we present herein for the first time that HACE1 is a key regulator of the Ub-selective autophagy pathway. Moreover HACE1’s functions in selective autophagy is independent of its E3 Ub ligase activity, but via protein–protein interactions mediated by its ANK domain. We propose that HACE1 could be the missed master regulator in the control of autophagic degradation of damaged organelle and proteins. Our in vivo studies demonstrate that HACE1 is a novel critical regulator of cardiac hypertrophy and remodelling. Our findings that HACE1 is upregulated in cardiac tissue of heart failure patients both make it an attractive candidate as a potential diagnostic biomarker for heart failure and provide an insight into the mechanisms of cardiac remodelling. Detection of HACE1 mRNA The collection and use of human samples in this study were approved by the Research Ethics Board of University Health Network and informed consent was obtained from patients/family members. HACE1 mRNA expression in human and mouse samples was detected by quantitative real-time reverse transcriptase (RT)–PCR analyses using standard procedures. Isolation of total RNA was performed using the Trizol reagent (Invitrogen). cDNAs were synthesized from 1 μg total RNA with the SuperScript III First-Strand Synthesis System for RT–PCR (Invitrogen) according to the manufacturer’s instructions. Quantitative RT–PCR was done using SYBR green assays (Roche Applied Science) with HACE1 -specific primers and both HPRT and GAPDH as an endogenous control. Real-time PCR reactions were carried out in 384-well plates using a Roche-LightCycler 480 System. All primer sequences are listed in Supplementary Table 2 . Mice strains and creation of pressure overload mouse model Hace1 -null mice with a mixed B6;129Ola genetic background were generated as reported previously [12] , subsequently backcrossed to C57BL/6J mice (Jackson Laboratory) for more than six generations and used for all the experiments reported in this study. GFP-LC3#53 transgenic mice [21] were imported from RIKEN Bio-Resource Center and were crossed with Hace1 −/− . mice to generate Hace1 −/− / GFP-LC3 Tg or Hace1 +/+ / GFP-LC3 Tg mice. Mice were genotyped by PCR [12] and maintained at the Animal Resources Centre of the University Health Network. All animal experimental protocols were approved by the Animal Care and Use Committee of the University Health Network and performed in accordance with the institutional guidelines. Male Hace1 −/− and Hace1 +/+ mice (15–17-week old) with body weight from 27 to 29 g were subjected to pressure overload by sTAC as previously described [13] . In brief, mice were anaesthetized with ketamine (IP; 90 mg kg −1 ) and Rompun (IP; 10 mg kg −1 ). The chest was opened, and a horizontal skin incision was made at the level of the two to three intercostal space. The start of the descending aorta was identified right after the subclavian branch. A 7-0 silk suture was placed around the beginning of the descending aorta and tied around a 27-gauge blunt needle, which was subsequently removed. At the end of the procedure, the chest and skin were closed. The mice were kept on a heating pad until responsive to stimuli. Sham-operated animals underwent the identical procedure, except that the aortic constriction was not placed. The integrity of the sTAC operation was confirmed by measuring the systolic pressure gradient shortly after the operation, which generated a systematic increase in systolic pressure from sham- (78 mm Hg) to sTAC (170 mm Hg) -operated heart. Owing to the high early mortality rate of the Hace1 −/− mice post sTAC, the experiment was only carried out for 4 days. Cardiac function evaluation Cardiac function was evaluated prior to sTAC and at day 2 and day 4 after sTAC using echocardiography as described previously 2. In brief, mice were sedated with 1% isoflurane/oxygen, and echocardiographic images were recorded using an Acuson Sequoia C256 System (Siemens Medical Solutions) with a 15L8 transducer. Depth and frequency were set at 2 cm and 13 MHz, respectively. The heart was first imaged in 2D mode in the parasternal short-axis view. From this view, an M-mode cursor was positioned perpendicular to the interventricular septum and posterior wall of the Left ventricular (LV) at the level of the papillary muscles, and M-mode images were obtained for measurement of wall thickness and chamber dimensions with the use of the leading-edge convention adapted by the American Society of Echocardiography. LV end-diastolic dimension (LVEDD) and LV end-systolic dimension (LVESD) were measured; percentage of LV fractional shortening (%FS) was described as [(LVEDD-LVESD)/(LVEDD) × 100%]. Histology, immunohistochemistry and TEM For morphometry, hearts were arrested in diastole with 1 M KCl, fixed with neutral buffered 10% formalin solution (Sigma HT501128), embedded in paraffin and sectioned to a thickness of 5 μm. Haematoxylin and eosin-stained sections were used for measurement of heart morphology and cardiomyocyte cross-sectional area using SimplePCI version 6 image analysis software (Hamamatsu Corporation). For immunohistochemistry, samples were fixed with buffered 4% paraformaldehyde, and paraffin sections were performed with minimal antigen retrieval (0.3% Triton X-100) using the following antibodies: mono- and polyubiquitinylated conjugates (FK2) (Enzo Life Science, PW8810, 1:100), p62 (Progen, GP62C, 1:100), GFP (Life Technologies, G10362, 1:200). Following overnight incubation with primary antibody, the sections were incubated with a matching biotinylated secondary antibody and detected by using VECTASTAIN ABC (peroxidase) system (Vector Labs). Negative controls were performed for all immunostaining by omission of the primary antibody. For TEM analysis, fresh isolated LV were minced into 1–2 mm 3 cubes and fixed with 2% glutaraldehyde in 0.1 M cacodylate buffer for 1 h at room temperature. Finally, the tissue was cut into 70 nm sections with an ultramicrotome, placed on TEM grids and imaged with a FEI Tecnai TEM operated at 80 kV at the Pathology Laboratory of the Hospital for Sick Children according to standard procedures. Immunoblotting Whole-cell lysates from tissue and cell samples were prepared on ice with cell lysis buffer (Cell Signaling, 9803) containing a Complete cocktail of proteases inhibitors (Roche Applied Science, 05892791001). Lysates were cleared by centrifugation at 12,000 r.p.m. for 10 min. The supernatants were collected and protein concentrations determined using the Bio-Rad Bradford protein assay kit (Bio-Rad). Twenty micrograms of protein lysate was separated by NuPAGE SDS–PAGE Gel System (Life Technologies) and electrophoretically transferred to polyvinylidene difluoride membranes (Invitrogen). Membranes were incubated overnight at 4 °C with antibodies reactive to the following proteins: ubiquitin (P4D1) (Cell Signaling, 3936, 1:1,000), p62 (Progen, GP62C, 1:1,000), LC3 (Novus, NB100-2331, 1:500), GFP (Life Technologies, A11121), HA (Monoclonal Antibody Facility, Hospital for Sick Children, 12CA5, 1:1,000), Unc-45b (GenWay, EV0087,1:1,000), gelsolin (BD, 610412, 1:1,000), vimentin (R28) (Cell Signaling, 3932, 1:1,000), Fhl1 (Novus, NB100-1461, 1:1,000) vinculin (Sigma, V4505, 1:1,000), β-tubulin (Sigma, T8328, 1:1,000), caldesmon (Abcam, ab32330, 1:1,000), Hsc70 (Abcam, ab2788, 1:1,000), Hsp70 (Stressgen, SPA810, 1:1,000), Hsp25 (Stressgen, SPA801, 1:1,000), connexin 40 (Life Technologies, 36-5000, 1:1,000) and connexin 43 (Life Technologies, 71-0700, 1:1,000). Blots were incubated with horseradish peroxidase-conjugated goat anti-mouse IgG (Bio-Rad, 170-5046, 1:50,000), goat anti-rabbit IgG (Bio-Rad, 170-5047, 1:100,000), monoclonal mouse anti-goat IgG (Jackson ImmunoResearch, 205-032-176, 1:50,000) or goat anti-guinea pig IgG (Jackson ImmunoResearch, 106-035-003, 1:100,000) and developed using ECL or ECL Plus Western Blotting Detection System (Amersham Biosciences). To normalize signals to total protein, blot membranes were stripped and re-probed with antibody against Gapdh (Cell Signaling, 2118, 1:2,000). The quantification of signals was performed by densitometry of scanned autoradiographs with the aid of Quantity One software (version 4.6; Bio-Rad). Proteasome activities were measured by the Chemicon Proteasome Activity Assay Kit (Millipore, APT280). In brief, freshly harvested heart samples were lysed in lysis buffer (50 mM HEPES (pH 7.5), 5 mM EDTA, 150 mM NaCl and 1% Triton X-100) supplemented with 2 mM ATP and were cleared by centrifuge at 15,000 r.p.m. for 20 min at 4 °C. Equal amounts of protein (determined by Bio-Rad Bradford protein assay) were used for preparing assay mixtures in a 96-well fluorometer plate and the remaining steps were conducted following the manufacturer’s instruction. Fluorescence data were collected using a Molecular Devices Spectra Max M5 plate reader using 380 nm excitation and 460 nm emission. Culture of mouse neonatal ventricular cardiomyocytes Cell culture of neonatal mouse cardiomyocytes was prepared from newborn Hace1 −/− and WT mouse hearts within 48 h of birth. In brief, after trimming, left ventricles were mechanically minced in Ca 2+ - and Mg 2+ -free Hank’s balanced salt solution (HBSS) on ice, and then subjected to stepwise enzymatic digestion with 0.15% trypsin (Invitrogen) in disassociation solution (137 mmol l −1 NaCl, 5.36 mmol l −1 KCl, 0.81 mmol l −1 MgSO 4, 5.55 mmol l −1 dextrose, 0.44 mmol l −1 KH 2 PO 4, 0.34 mmol l −1 Na 2 HPO 4 7H 2 O and 20.06 mmol l −1 HEPES, pH 7.4). Cells released after the first digestion were discarded, whereas cells from subsequent digestion were transferred into GIBCO DMEM/F-12 medium (Invitrogen) supplemented with 10% fetal bovine serum (FBS; Invitrogen) until all cardiac cells were isolated (~5 times). The resulting mixture was centrifuged for 5 min at 800 r.p.m., resuspended in DMEM/F-12 medium and preplated for 2 h to remove non-cardiomyocytes based on the observation that non-muscle cells attach to the substrata more rapidly. The cardiomyocytes were then collected and plated on laminin-coated culture plates at a density of 2 × 10 6 cells ml −1 in DMEM/F-12 plus 10% FBS and 0.1 μM 5-bromodeoxyuridine (to inhibit growth of non-myocytes). Cells were incubated at 37 °C with 5% CO 2 in a humidified atmosphere. A confluent monolayer of spontaneously beating cardiomyocytes was formed within 2 days and was ready for downstream gene transfer and treatment. Protein aggregate clearance assay Protein aggregate clearance assays were performed with both neonatal NCMs and MEF cell culture. MEF cells were prepared from hace1 −/− or littermate WT E13.5 mouse embryos and were grown in DMEM (Invitrogen) containing 10% FBS (Invitrogen), 10 units ml −1 penicillin (Invitrogen) and 0.1 μg ml −1 streptomycin (Invitrogen). Hace1 −/− MEF stably expressing WT HACE1, C876S E3 ligase dead mutant ( HACE1C876S ) and empty vector were generated using a retroviral system as described previously [11] . The three GFP-tagged HACE1 plasmids used for transient transfection into hace1 −/− MEF were from OriGene; pCMV-AC-HACE1-GFP (RG205602), HACE1ΔHECT and HACE1ΔAN were generated by gene synthesis and subcloned into pCMV-AC-mGFP plasmid (OriGene). For protein aggregate clearance assay, MEF cells were grown on Millicell EZ slides (Millipore) to about 70% confluence and were treated with 10 μg ml −1 puromycin (Sigma, P8833) for 4 h to induce ubiquitinated protein aggregate formation, followed by extensive washing. Aggregate clearance was followed for a further 8 h (total 12 h) incubation with fresh medium. Non-treated MEFs were used as negative controls. After treatment, MEF were washed three times in PBS, followed by fixing in 4% paraformaldehyde and were subjected to fluorescence staining for Ub-conjugated protein with an anti-FK2 antibody (Enzo Life Science, PW8810, 1:100). In brief, fixed cells on the slides were first permeabilized for 2 min in 0.1% Triton-X 100, and then blocked for 1 h in PBS with 3% normal goat serum and 1% BSA. Slides were next incubated overnight at 4 °C with FK2 antibody, followed by staining with Alexa Fluor 633 goat anti-mouse IgG (Life Technologies, A21052, 1:1,000) for 1 h. After being nuclei stained with Hoechst 33342 (Life Technologies, H1399), cells were mounted with ProLong Gold antifade reagent (Life Technologies, P-36934) and subjected to confocal examination on an Olympus FluoView 1000 Laser Scanning Confocal Microscope. The total fluorescence intensity from the FK2 staining was measured using Olympus Fluoview FV1000 viewer software. Small interference RNA and p62 immunoprecipitation Knockdown of p62 in Hace1 +/+ and Hace1 −/− NCMs was achieved using ON-TARGET plus SMARTpool mouse Sqstm1 (p62) siRNAs (Thermo/Dhamacon l-047628-01); ON-TARGET plus non-targeting siRNA pool (D-001810-01) were used as control. DharmaFECT 1 Transfection Reagent (T-2001) was used to transfect siRNAs in a final concentration of 20 nM to NCM cells and knockdown of p62 mRNA was confirmed by RT–PCR using p62 gene-specific primers. Forty-eight hours after knockdown, cells were subjected to protein aggregate clearance assay as illustrated in the above section. p62 immunoprecipitation was performed by using Pierce Classic Magnetic IP/Co-IP kit (Thermo Scientific, 88804) with guinea pig polyclonal anti-p62 (Progen, GP62C 1:100) as IP antibody; and the pull-down products were analysed by western blot with anti-mono and polyubiquitin-conjugated antibody (FK2) (Enzo Life Sciences, BML-PW01510, 1:1,000). Plasmid transfection and microscopy Transient transfection of plasmid constructs into both primary mouse NCM and MEF was carried out by using the Transfection Reagent Xfect (Clontech, 631318) or a Neon Transfection System (Life Technologies) according to standard protocols. HACE1 expression plasmids pCMV6-AC-HACE1-GFP and pCMV6-AC-HACE1-RFP were from OriGene. The tandem tagged mRFP-GFP-LC3 reporter ( tfLC3 ) plasmid was from Addgene. Forty-eight hours after transfection, cells were treated with either 10 μg ml −1 puromycin or 1 μM MG132 with or without 100 nM Baf for the indicated time, followed by washing three times in PBS. Cells were then fixed in 4% paraformaldehyde, permeabilized for 2 min in 0.1% Triton-X 100 and then blocked for 1 h in PBS with 3% normal goat serum and 1% BSA. For the tandem tagged mRFP-GFP-LC3 reporter assay, cells were mounted with ProLong Gold antifade reagent with 4',6-diamidino-2-phenylindole (Invitrogen, P-36931) and subjected to confocal examination on an Olympus FluoView 1,000 Laser Scanning Confocal Microscope. Co-localization efficiency of mRFP with GFP signals of tfLC3 puncta was measured using ImageJ software, and has been shown as the percentage of the total number of mRFP puncta. For HACE1 co-localization with p62 and Lamp1, an immunostaining step with anti-p62 (Progen, GP62C) and anti-Lamp1 antibody (C-20) (Santa Cruz Biotech) was added before confocal examining. For HA-HACE1 co-localization with Ub + protein aggregates, HA-HACE1 was detected with an anti-HA mouse IgG1 monoclonal antibody prelabelled with the Zenon Alexa Fluor 488 Mouse IgG1 Labeling Kit (Life Technologies, Z-25002); Ub-conjugated proteins were labelled using an anti-FK2 antibody (Enzo Life Science, PW8810, 1:100), followed by staining with Alexa Fluor 633 goat anti-mouse IgG (Life Technologies, A21052,1:1,000). Fluorescence microscopy was carried out on a Nikon Eclipse TE2000-U. Generation of HACE-expressing MEF and immunoprecipitation Hace1 −/− MEF stably expressing an N-terminal HA-tagged full-length human HACE1 cDNA ( HA-HACE1 ) was generated using a retroviral system as described previously [11] . In brief, HA-tagged HACE1 cDNA was generated by subcloning the HACE1 coding region from the IMAGE cDNA clone number 4838835 (ATCC; GenBank accession number BC034982) into mammalian expression vector pcDNA3-HA (Life Technologies). The HA-tagged Cys to Ser mutant (C876S) form of HACE1 was generated by Site directed mutagenesis using the QuickChange kit (Stratagene). HA-tagged HACE1 cDNA was subsequently subcloned into pMSCV- hygromycin vector (Clontech) followed by transfection into the BOSC23 ecotropic retroviral packaging cell line using calcium phosphate precipitation. Retrovirus-containing supernatants were collected 48 h after transfection and used to infect Hace1 −/− MEF. To generate stably transfected MEF cells, infected cells were selected using 200 μg ml −1 hygromycin (Life Technologies) for 48 h. The HACE1 immunoprecipitation (IP) analysis was performed using anti-HA Affinity Matrix (Roche Applied Science, 11 815 016 001); for Unc-45b IP, immunoprecipitation kit (Protein G) (Roche Applied Science, 11 719 836 001) with goat polyclonal anti Unc-45b (GenWay, EV0087, 1:50) as IP antibody. Equal amounts of cell lysate were immunoprecipitated with anti-HA or anti-Unc-45b and were subjected to SDS–PAGE and immunoblotted with the indicated antibodies. To confirm that HACE1 is also binding to the same proteins as in the heart, the anti-HA Affinity Matrix that has been incubated with HA-HACE1 MEF or control MSCV MEF lysates was further incubated with whole-heart lysate (Co-Co-IP) from HACE1 WT mice and equal amounts of eluate were subjected to immunoblotting with the indicated antibodies. MS analysis To map out the molecular interaction of HACE1, we examined the anti-HA Co-IP products by MS analysis, essentially as previously described [41] , [48] . In brief, samples were subjected to an in-solution tryptic digestion and then subjected to solid-phase extraction using OMIX C-18 pipette tips (Varian Inc.). MS experiments were carried out on a LTQ linear ion-trap mass spectrometer (Thermo Fisher Scientific) equipped with a nanoelectrospray source (Proxeon Biosystems, Denmark). Peptides were eluted from the microcapillary columns using a 2-h gradient as described [41] . Spectra were identified by converting Raw MS files to m/z XML using ReAdW and searched by a locally installed version of X!Tandem against a mouse IPI (International Protein Index; http://www.ebi.ac.uk/IPI ) protein sequence database created on August 2010. To estimate and minimize our false-positive rate, the protein sequence database also contained every IPI protein sequence in its reversed amino-acid orientation (target-decoy strategy) as recently described [41] , [48] . In this study we set the value of total reverse spectra to total forward spectra to 0.5%, resulting in a low number of decoy sequences in the final output. Only peptides matching these criteria were accepted to generate the final list of identified proteins, with further criteria set to select only those proteins identified with a minimum of two unique peptides. Statistical analysis For all multiple comparisons of normally distributed data, one-way analysis of variance followed by Bonferroni’s multiple comparison post-tests were used, while for comparison of two groups of normally distributed data as shown in Fig. 1b , unpaired two-tailed Student’s t -tests were used. Survival rates were analysed by the Kaplan–Meier method, and difference between groups was tested with the log-rank χ 2 -test. Statistical analyses were conducted using GraphPad Prism 5 software. All values are presented as means±s.e.m. ; n refers to the sample size. P <0.05 was considered significant. How to cite this article: Zhang, L. et al. HACE1-dependent protein degradation provides cardiac protection in response to haemodynamic stress. Nat. Commun. 5:3430 doi: 10.1038/ncomms4430 (2014).